Surrogate reporter-based enrichment of cells containing RNA-guided Cas9 nuclease-induced mutations RNA-guided endonucleases (RGENs), which are based on the clustered, regularly interspaced, short palindromic repeat (CRISPR)-CRISPR-associated (Cas) system, have recently emerged as a simple and efficient tool for genome editing. However, the activities of prepared RGENs are sometimes low, hampering the generation of cells containing RGEN-induced mutations. Here we report efficient methods to enrich cells containing RGEN-induced mutations by using surrogate reporters. HEK293T cells are cotransfected with the reporter plasmid, a plasmid encoding Cas9 and a plasmid encoding crRNA and tracrRNA, and subjected to flow cytometric sorting, magnetic separation or hygromycin selection. The selected cell populations are highly enriched with cells containing RGEN-induced mutations, by a factor of up to 11-fold as compared with the unselected population. The fold enrichment tends to be high when RGEN activity is low. We envision that these reporters will facilitate the use of RGEN in a wide range of biomedical research. RNA-guided endonucleases (RGENs)—programmable nucleases derived from the RNA-guided CRISPR/Cas DNA cleavage system found in bacteria and archaea [1] , [2] —are emerging as a promising tool for targeted genome editing [3] , [4] , [5] , [6] , [7] , [8] , [9] , [10] . As part of their adaptive immune system, bacteria and archaea integrate short fragments (~20 bp) of invading foreign DNAs, termed ‘protospacers’, into their genomes at sites called CRISPRs (clustered regularly interspaced short panlindromic repeats) [2] . Three types of CRISPR systems have been identified; type II systems have been utilized for genome editing [3] , [4] , [5] , [6] , [7] , [8] , [9] , [10] . In such systems, the protospacers in the CRISPR are transcribed to give rise to pre-CRISPR RNA, which is subsequently processed to CRISPR RNA (crRNA) by RNase III. When CRISPR-associated protein 9 (Cas9) is complexed with crRNA and tracrRNA, it forms a sequence-specific endonuclease that recognizes the sequence complementary to that of crRNA and makes double-strand breaks. RGENs can be simplified by replacing crRNA and tracrRNA with a single-chain guide RNA (sgRNA) generated by combining crRNA and tracrRNA [3] . Genome editing using RGENs has been recently reported in various cell types and species such as bacteria [9] , plants [11] , [12] , [13] , C. elegans [6] , fruit flies [7] , zebrafish [8] , rats [14] , [15] , mice [5] , [15] , [16] and human cells [4] , [5] , [10] , [17] , including human pluripotent stem cells [10] , [18] , [19] . However, not all designed RGENs exhibit high activity [4] , [5] , [6] , [7] , [8] , [10] , [11] , [12] , [13] , [14] , [15] , [16] , [17] , [18] , hampering their use for genome engineering. Thus, simple methods for enriching cells containing RGEN-induced mutations would facilitate the use of this tool. If nuclease-induced mutations confer selective advantages on the cells, these modified cells can be enriched [20] . However, this approach cannot be applied to most genes whose disruption does not contribute to discernible phenotypes for selection. Gene-modified cells are often enriched by selecting cotransfected cells; for example, transcription activator-like effector nuclease (TALEN)-modified cells have been enriched by selecting transfected cells via flow cytometric sorting or antibiotic selection using vectors expressing fluorescent proteins or antibiotic resistance factors [21] , [22] , [23] . However, even in the transfected cells, nuclease-induced genome editing often occurs only in a limited fraction [24] . Thus, a method to select cells with high programmable nuclease activity would be an efficient approach to enrich cells with nuclease-induced mutations. We and others have previously observed that, when a target sequence on a chromosome was mutated by zinc finger nucleases (ZFNs), the same target sequence on the other homologous chromosome in the same cell is mutated more frequently than that in other cells [25] , [26] . This observation led us to postulate that an episomal surrogate reporter that contains the target sequence might faithfully reflect the nuclease’s activity on the chromosome in the same cell. This hypothesis was validated as we previously showed that surrogate reporters, together with flow cytometry, magnetic separation or hygromycin selection, can enable enrichment of cells containing mutations induced by two other types of engineered nucleases, ZFNs and TALENs [24] , [27] . RGENs differ from ZFNs and TALENs in several key respects. For example, both ZFNs and TALENs (which function as heterodimers) are composed solely of protein, whereas RGENs (which function as monomers) consist of protein and RNA. As a result, ZFNs and TALENs recognize target sequences via DNA–protein interactions, whereas RGENs do so by DNA–RNA interactions. Furthermore, the ZFN and TALEN catalytic domain is derived from the FokI nuclease, whereas the RGEN catalytic domain is from Cas9. Functionally, ZFNs (and probably TALENs) generate double-strand breaks in DNA with cohesive overhangs, whereas RGENs mainly lead to blunt ends. Given these unique features of RGENs, we examine whether cells containing RGEN-induced mutations can also be enriched with surrogate reporters. Here we show that three kinds of episomal surrogate reporters, coupled with flow cytometry, magnetic separation or hygromycin selection, can indeed enrich RGEN-induced mutant cells, which should facilitate the use of RGENs in biomedical research, medicine and biotechnology. Flow cytometric enrichment of cells containing mutations The reporter comprises an mRFP gene, an RGEN target sequence and two eGFP genes ( Fig. 1 ). To increase the sensitivity of the previously described fluorescent reporter [24] , we added another eGFP-encoding sequence at the end of the original eGFP sequence such that mutations of both (3n+1) and (3n+2) nucleotide insertions or deletions at the target sequence can lead to eGFP expression. In the absence of nuclease activity, the reporter-transfected cells will express only mRFP owing to the presence of double barriers: the two eGFP genes are both out of frame and the stop codon before the eGFP genes will terminate protein translation. If RGENs make double-strand breaks in the target sequence in the reporters, indels generated by error-prone nonhomologous end joining (NHEJ) can cause frame-shift mutations, rendering one of the eGFP genes expressed ( Fig. 1 ). To determine whether mutant cells can be enriched using flow cytometric reporters, we cotransfected a reporter plasmid, a plasmid encoding Cas9 and a plasmid encoding BMP1-targeting crRNA and tracrRNA into HEK293T cells. Twenty-four hours after the transfection, a considerable fraction of cells expressed mRFP, whereas a small fraction of cells expressed eGFP ( Supplementary Fig. 1 ), indicating that frame-shifting indels had already been generated at the target sequence by RGEN activity. In contrast, a previous study involving ZFNs showed that eGFP expression was barely observed at day 1 after transfection [24] , suggesting that RGENs may work faster than ZFNs. This observation is compatible with a recent report that RGEN-mediated gene editing can be detectable at ~20 h post transfection compared with ~40 h for TALENs [10] . The number of eGFP-expressing cells also gradually increased over 3 days, suggesting that RGEN activity was also present after 24 h post transfection. 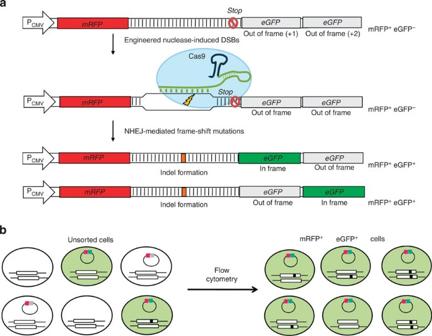Figure 1: Overview of flow cytometric enrichment of cells containing RGEN-induced mutations. (a) The working mechanism of the fluorescent reporter. mRFP is constitutively expressed by the CMV promoter (PCMV), whereas eGFP is not expressed without RGEN activity because the eGFP sequence is out of frame and there is a stop codon before eGFP. If a double-strand break (DSB) is introduced into the target sequence by an RGEN, the break is repaired by error-prone nonhomologous end joining (NHEJ), which often results in indels. This indel formation can cause frame shifts, making either of the eGFP genes in frame and expressed. (b) A schematic illustrating the enrichment of mutant cells in the mRFP+eGFP+cell population using flow cytometry. Reporter plasmids, chromosomal target loci and sites of mutations, represented by black boxes, are shown. Figure 1: Overview of flow cytometric enrichment of cells containing RGEN-induced mutations. ( a ) The working mechanism of the fluorescent reporter. mRFP is constitutively expressed by the CMV promoter (P CMV ), whereas eGFP is not expressed without RGEN activity because the eGFP sequence is out of frame and there is a stop codon before eGFP. If a double-strand break (DSB) is introduced into the target sequence by an RGEN, the break is repaired by error-prone nonhomologous end joining (NHEJ), which often results in indels. This indel formation can cause frame shifts, making either of the eGFP genes in frame and expressed. ( b ) A schematic illustrating the enrichment of mutant cells in the mRFP + eGFP + cell population using flow cytometry. Reporter plasmids, chromosomal target loci and sites of mutations, represented by black boxes, are shown. Full size image Three days after transfection, 9.4% of the cells were mRFP + eGFP + cells; these cells were flow cytometrically separated ( Fig. 2a ). To measure the RGEN-induced mutation frequencies (or indel %), we isolated genomic DNA and performed a T7 endonuclease I (T7E1) assay [26] , [28] . T7E1 recognizes and cleaves heteroduplexes formed by the hybridization of wild-type and mutant DNA sequences. This assay showed that the mutation frequency at the BMP1 gene in mRFP + eGFP + cells was 41%, 18-fold higher than that in unsorted cells (2.3%) ( Fig. 2b ), indicating drastic enrichment of BMP1-mutated cells. Comparable mutation frequencies were obtained in cells transfected with only Cas9 and guide RNAs (3.3%), unsorted cells (2.3%) and mRFP + eGFP − cells (2.9%), which is in line with previous observations using ZFNs [24] . When we determined the DNA sequences around the target site, we found that the mutation frequency in the flow cytometrically sorted mRFP + eGFP + cells was 33%, 7.4-fold higher than that in unsorted cells (4.5%), corroborating the efficient enrichment of cells containing RGEN-induced mutations ( Fig. 2c ). 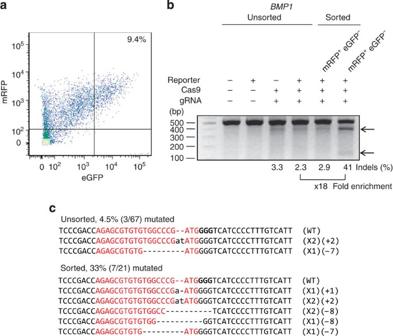Figure 2:Flow cytometric enrichment ofBMP1-disrupted cells. (a) Flow cytometry of HEK293T cells at 3 days after cotransfection of the reporter plasmid, a plasmid encoding Cas9 and a plasmid encodingBMP1-targeting crRNA and tracrRNA. The percentage of mRFP+eGFP+cells is shown. (b) The frequency of RGEN-induced mutations as determined by the T7E1 assay. Arrows indicate the expected positions of DNA bands cleaved by mismatch-sensitive T7E1. The numbers at the bottom of the gel indicate mutation percentages calculated by band intensities. (c) DNA sequences of the wild-type (WT) and mutant clones, with RGEN recognition sites shown in red and the protospacer adjacent motif (PAM) sequence in bold characters. Dashes and lower-case letters indicate deleted and inserted bases, respectively (the number of inserted or deleted bases are described in the parentheses; out-of-frame and in-frame mutations are indicated using red and black colours, respectively). The number of occurrences is shown in parentheses; X1 and X2 indicates the number of each clone. Mutation frequencies were obtained by dividing the number of mutant clones by the number of total clones. Figure 2: Flow cytometric enrichment of BMP1 -disrupted cells . ( a ) Flow cytometry of HEK293T cells at 3 days after cotransfection of the reporter plasmid, a plasmid encoding Cas9 and a plasmid encoding BMP1 -targeting crRNA and tracrRNA. The percentage of mRFP + eGFP + cells is shown. ( b ) The frequency of RGEN-induced mutations as determined by the T7E1 assay. Arrows indicate the expected positions of DNA bands cleaved by mismatch-sensitive T7E1. The numbers at the bottom of the gel indicate mutation percentages calculated by band intensities. ( c ) DNA sequences of the wild-type (WT) and mutant clones, with RGEN recognition sites shown in red and the protospacer adjacent motif (PAM) sequence in bold characters. Dashes and lower-case letters indicate deleted and inserted bases, respectively (the number of inserted or deleted bases are described in the parentheses; out-of-frame and in-frame mutations are indicated using red and black colours, respectively). The number of occurrences is shown in parentheses; X1 and X2 indicates the number of each clone. Mutation frequencies were obtained by dividing the number of mutant clones by the number of total clones. Full size image Next, to determine whether this reporter system is applicable to other RGENs, we tested both F13A1 and PPP1R1B -targeting RGENs. Three days after cotransfecting F13A1- and PPP1R1B -targeting RGEN and reporter plasmids, 8.2 and 7.8% of HEK293T cells were mRFP + eGFP + cells ( Fig. 3a,d ). Following the isolation of genomic DNA from the sorted cells, the T7E1 assay revealed that the mutation frequencies in these cells were 36% and 53%, respectively, which is 7.8- and 4.6-fold higher than in unsorted cells ( Fig. 3b,e ), suggesting that reporter-based flow cytometric sorting is portable to other RGENs for the enrichment of mutant cells. This enrichment was also validated by sequencing the genomic DNA around the target site, which revealed that the mutation frequency after F13A1 and PPP1R1B -targeting RGEN treatment was 10-fold (32%) and 4.3-fold (23%) higher, respectively, in mRFP + eGFP + cells than in unsorted cells ( Fig. 3c,f ). In line with the result with BMP1 -targeting RGENs, the mutation frequencies of cells transfected with only Cas9 and guide RNAs without the reporter plasmid, unsorted cells and mRFP + eGFP − cells were all comparable (in the F13A1 group, 5.0%, 4.6% and 5.2%, respectively; in the PPP1R1B group, 11%, 11% and 12%, respectively). We next tested this reporter system using HeLa cells, a human cervical cancer cell line. Flow cytometry showed that 6.7% of these cells were mRFP + eGFP + and the T7E1 assay revealed that the mutation frequency in the sorted cells was 52%, 4.5-fold higher than in unsorted cells ( Supplementary Fig. 2 ), suggesting that this flow cytometric sorting is also applicable to other cell types for the enrichment of cells containing RGEN-induced mutations. 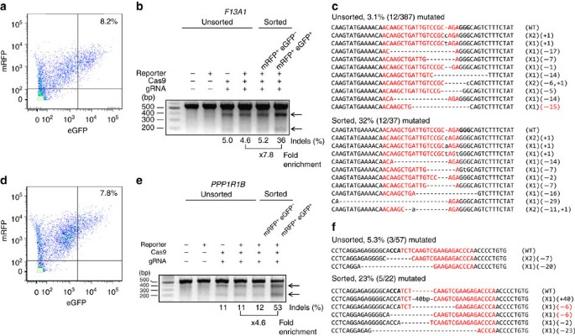Figure 3:Flow cytometric enrichment ofF13A1andPPP1R1B-disrupted cells. Three days after cotransfection of the reporter plasmid, a plasmid encoding Cas9 and a plasmid encodingF13A1-(a–c) andPPP1R1B– (d–f) targeting crRNA and tracrRNA, HEK293T cells were flow cytometrically sorted and analysed. (a,d) Flow cytometry; the percentage of mRFP+eGFP+cells is shown. (b,e) The frequency of RGEN-induced mutations as determined by the T7E1 assay is shown. Arrows indicate the expected positions of DNA bands cleaved by mismatch-sensitive T7E1. The numbers at the bottom of the gel indicate mutation percentages calculated by band intensities. (c,f) DNA sequences of the wild-type (WT) and mutant clones, with RGEN recognition sites shown in red and the protospacer adjacent motif (PAM) sequence in bold characters. Dashes and lower case letters indicate deleted and inserted bases, respectively (the number of inserted or deleted bases are described in the parentheses; out-of-frame and in-frame mutations are indicated using red and black colours, respectively). The number of occurrences is shown in parentheses; X1 and X2 indicate the number of each clone. Mutation frequencies were obtained by dividing the number of mutant clones by the number of total clones. Figure 3: Flow cytometric enrichment of F13A1 and PPP1R1B -disrupted cells . Three days after cotransfection of the reporter plasmid, a plasmid encoding Cas9 and a plasmid encoding F13A1- ( a – c ) and PPP1R1B – ( d – f ) targeting crRNA and tracrRNA, HEK293T cells were flow cytometrically sorted and analysed. ( a , d ) Flow cytometry; the percentage of mRFP + eGFP + cells is shown. ( b , e ) The frequency of RGEN-induced mutations as determined by the T7E1 assay is shown. Arrows indicate the expected positions of DNA bands cleaved by mismatch-sensitive T7E1. The numbers at the bottom of the gel indicate mutation percentages calculated by band intensities. ( c , f ) DNA sequences of the wild-type (WT) and mutant clones, with RGEN recognition sites shown in red and the protospacer adjacent motif (PAM) sequence in bold characters. Dashes and lower case letters indicate deleted and inserted bases, respectively (the number of inserted or deleted bases are described in the parentheses; out-of-frame and in-frame mutations are indicated using red and black colours, respectively). The number of occurrences is shown in parentheses; X1 and X2 indicate the number of each clone. Mutation frequencies were obtained by dividing the number of mutant clones by the number of total clones. Full size image Magnetic separation-mediated enrichment of mutant cells We next tested whether magnetic separation can enrich cells containing RGEN-induced mutations. For this experiment, we used magnetic reporters [27] , in which both eGFP and H-2K k are expressed by frame-shifting indel formation in the target sequence of the reporter ( Supplementary Fig. 3 ). Three days after the cotransfection of the reporter plasmid, a plasmid encoding Cas9 and a plasmid encoding F13A1 -targeting crRNA and tracrRNA into HEK293T cells ( Supplementary Fig. 4 ), we isolated H-2K k expressing cells by magnetic separation using a magnetic bead-conjugated anti-H2K k antibody. Twenty-four hours after these cells were plated into dishes, fluorescent microscopic observation showed that the population of magnetically separated cells was enriched with eGFP + cells ( Fig. 4a ), suggesting enrichment of cells containing RGEN-induced indels at the target site. The T7E1 assay revealed that the mutation frequency in the magnetically separated cells was 55%, 9.6-fold higher than that in unseparated cells (5.7%) ( Fig. 4b ), indicating efficient enrichment of cells containing RGEN-induced F13A1 mutations. The mutation frequencies of cells transfected with only Cas9 and guide RNAs without the reporter plasmid, unsorted cells and mRFP + eGFP − cells were all similar (6.4%, 5.7% and 6.7%, respectively). Sequencing the genomic DNA around the target site after PCR amplification revealed that the mutation frequency in the magnetically separated cells was 31%, 11-fold higher than in the unseparated cells (2.8%) ( Fig. 4c ), corroborating the drastic enrichment of mutant cells mediated by magnetic separation. 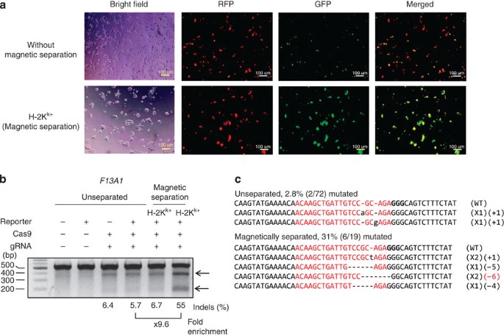Figure 4:Magnetic separation-mediated enrichment ofF13A1-disrupted cells. (a) Fluorescent microscopy of HEK293T cells cultured for 1 day after magnetic separation, which was performed 3 days after cotransfection of the reporter plasmid, a plasmid encoding Cas9 and a plasmid encodingF13A1-targeting crRNA and tracrRNA. Magnetic separation enriched eGFP+cells. Scale bar, 100 μm. (b) The frequency of RGEN-induced mutations as determined by the T7E1 assay is shown. Arrows indicate the expected positions of DNA bands cleaved by mismatch-sensitive T7E1. The numbers at the bottom of the gel indicate mutation percentages calculated by band intensities. (c) DNA sequences of the wild-type (WT) and mutant clones, with RGEN recognition sites shown in red and the protospacer adjacent motif (PAM) sequence in bold characters. Dashes and lower case letters indicate deleted and inserted bases, respectively (the number of inserted or deleted bases are described in the parentheses; out-of-frame and in-frame mutations are indicated using red and black colours, respectively). The number of occurrences is shown in parentheses; X1 and X2 indicates the number of each clone. Mutation frequencies were obtained by dividing the number of mutant clones by the number of total clones. Figure 4: Magnetic separation-mediated enrichment of F13A1 -disrupted cells . ( a ) Fluorescent microscopy of HEK293T cells cultured for 1 day after magnetic separation, which was performed 3 days after cotransfection of the reporter plasmid, a plasmid encoding Cas9 and a plasmid encoding F13A1 -targeting crRNA and tracrRNA. Magnetic separation enriched eGFP + cells. Scale bar, 100 μm. ( b ) The frequency of RGEN-induced mutations as determined by the T7E1 assay is shown. Arrows indicate the expected positions of DNA bands cleaved by mismatch-sensitive T7E1. The numbers at the bottom of the gel indicate mutation percentages calculated by band intensities. ( c ) DNA sequences of the wild-type (WT) and mutant clones, with RGEN recognition sites shown in red and the protospacer adjacent motif (PAM) sequence in bold characters. Dashes and lower case letters indicate deleted and inserted bases, respectively (the number of inserted or deleted bases are described in the parentheses; out-of-frame and in-frame mutations are indicated using red and black colours, respectively). The number of occurrences is shown in parentheses; X1 and X2 indicates the number of each clone. Mutation frequencies were obtained by dividing the number of mutant clones by the number of total clones. Full size image When we tested this magnetic reporter using BMP1 - and PPP1R1B -targeting RGENs, the T7E1 assay showed that the mutation frequency was 42% and 60% in magnetically separated cells, respectively, which is 16- and 3.7-fold higher than in unseparated cells (2.6% and 16.5%, respectively) ( Fig. 5a,c ). This enrichment was confirmed by sequencing the target region, which revealed that the mutation frequency after BMP1 - and PPP1R1B -targeting RGEN treatment was 10-fold (32%) and 3.7-fold (26%) higher, respectively, in magnetically separated cells than in unseparated cells ( Fig. 5b,d ). This result indicates that cells in which mutations are induced by other RGENs can be efficiently enriched using magnetic reporters. Compatible with the result using F13A1 -targeting RGENs, the mutation frequencies of cells transfected with only Cas9 and guide RNAs without the reporter plasmid, unsorted cells and mRFP + eGFP − cells were all comparable (in the BMP1 group, 2.7%, 2.6% and 3.8%, respectively; in the PPP1R1B group, 16.1%, 16.5% and 16.7%, respectively). This magnetic separation-mediated enrichment of mutant cells was also validated in other cell types, as evidenced by 3.8-fold enrichment of HeLa cells containing RGEN-induced mutations, reaching a mutation frequency of 36% as calculated by the T7E1 assay ( Supplementary Fig. 5 ). 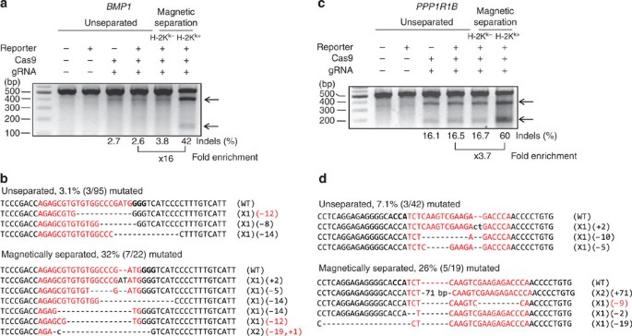Figure 5:Magnetic separation-mediated enrichment ofBMP1- andPPP1R1B-disrupted cells. Magnetic separation was performed 3 days after cotransfection of the reporter plasmid, a plasmid encoding Cas9 and a plasmid encodingBMP1- (a,b) orPPP1R1B- (c,d) targeting crRNA and tracrRNA into HEK293T cells. (a,c) The frequency of RGEN-induced mutations was determined by the T7E1 assay. Arrows indicate the expected positions of DNA bands cleaved by mismatch-sensitive T7E1. The numbers at the bottom of the gel indicate mutation percentages calculated by band intensities. (b,d) DNA sequences of the wild-type (WT) and mutant clones, with RGEN recognition sites shown in red and the protospacer adjacent motif (PAM) sequence in bold characters. Dashes and lower case letters indicate deleted and inserted bases, respectively (the number of inserted or deleted bases are described in the parentheses; out-of-frame and in-frame mutations are indicated using red and black colours, respectively). The number of occurrences is shown in parentheses; X1 and X2 indicate the number of each clone. Mutation frequencies were obtained by dividing the number of mutant clones by the number of total clones. Figure 5: Magnetic separation-mediated enrichment of BMP1 - and PPP1R1B -disrupted cells . Magnetic separation was performed 3 days after cotransfection of the reporter plasmid, a plasmid encoding Cas9 and a plasmid encoding BMP1 - ( a , b ) or PPP1R1B - ( c , d ) targeting crRNA and tracrRNA into HEK293T cells. ( a , c ) The frequency of RGEN-induced mutations was determined by the T7E1 assay. Arrows indicate the expected positions of DNA bands cleaved by mismatch-sensitive T7E1. The numbers at the bottom of the gel indicate mutation percentages calculated by band intensities. ( b , d ) DNA sequences of the wild-type (WT) and mutant clones, with RGEN recognition sites shown in red and the protospacer adjacent motif (PAM) sequence in bold characters. Dashes and lower case letters indicate deleted and inserted bases, respectively (the number of inserted or deleted bases are described in the parentheses; out-of-frame and in-frame mutations are indicated using red and black colours, respectively). The number of occurrences is shown in parentheses; X1 and X2 indicate the number of each clone. Mutation frequencies were obtained by dividing the number of mutant clones by the number of total clones. Full size image Mutant cell enrichment using hygromycin selection The separation methods discussed above require instruments such as flow cytometers and magnetic separators, and both necessitate trypsinization of adherent cells to make single-cell suspensions. However, antibiotic selection does not require any special instruments or antibodies. Thus, we attempted to enrich cells containing RGEN-induced mutations using antibiotic selection. For this approach, we used a hygromycin reporter [27] that expresses a hygromycin-resistance protein (Hygro R )–eGFP fusion protein only when frame-shifting indels are generated in the target sequences of the reporter by nuclease activity ( Supplementary Figs 6 and 7 ). Hygromycin treatment for 2 days starting at 2 days after the cotransfection of the reporter plasmid, a plasmid encoding Cas9 and a plasmid encoding PPP1R1B -targeting crRNA and tracrRNA resulted in the death of most cells; the remaining population of cells was enriched for eGFP + cells ( Fig. 6a ). The T7E1 assay showed that the mutation frequency at the PPP1R1B gene in the hygromycin-selected cells was 57%, 8.6-fold higher than that in unselected cells (6.6%) ( Fig. 6b ), indicating efficient enrichment of mutant cells. DNA sequencing of the region containing the target site confirmed this enrichment by revealing that the mutation frequency in the hygromycin-resistant cells was 23%, 7.7-fold higher than that in unselected cells ( Fig. 6c ). 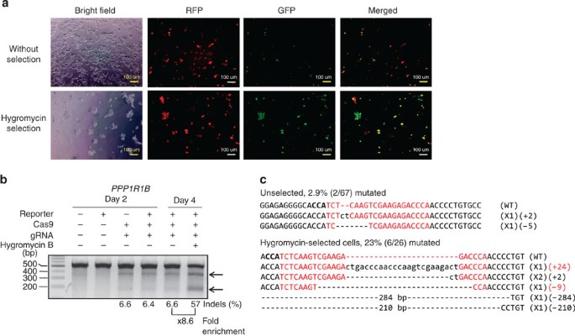Figure 6:Hygromycin selection-mediated enrichment ofPPP1R1B-disrupted cells. (a) Fluorescent microscopy of HEK293T cells treated with hygromycin for 2 days starting 2 days after the cotransfection of the reporter plasmid, a plasmid encoding Cas9 and a plasmid encodingPPP1R1B-targeting crRNA and tracrRNA. Hygromycin selection-enriched eGFP+cells. Scale bar, 100 μm. (b) The frequency of RGEN-induced mutations as determined by the T7E1 assay. Arrows indicate the expected positions of DNA bands cleaved by mismatch-sensitive T7E1. The numbers at the bottom of the gel indicate mutation percentages calculated by band intensities. (c) DNA sequences of the wild-type (WT) and mutant clones, with RGEN recognition sites shown in red and the protospacer adjacent motif (PAM) sequence in bold characters. Dashes and lower case letters indicate deleted and inserted bases, respectively (the number of inserted or deleted bases are described in the parentheses; out-of-frame and in-frame mutations are indicated using red and black colours, respectively). The number of occurrences is shown in parentheses; X1 and X2 indicates the number of each clone. Mutation frequencies were obtained by dividing the number of mutant clones by the number of total clones. Figure 6: Hygromycin selection-mediated enrichment of PPP1R1B -disrupted cells. ( a ) Fluorescent microscopy of HEK293T cells treated with hygromycin for 2 days starting 2 days after the cotransfection of the reporter plasmid, a plasmid encoding Cas9 and a plasmid encoding PPP1R1B -targeting crRNA and tracrRNA. Hygromycin selection-enriched eGFP + cells. Scale bar, 100 μm. ( b ) The frequency of RGEN-induced mutations as determined by the T7E1 assay. Arrows indicate the expected positions of DNA bands cleaved by mismatch-sensitive T7E1. The numbers at the bottom of the gel indicate mutation percentages calculated by band intensities. ( c ) DNA sequences of the wild-type (WT) and mutant clones, with RGEN recognition sites shown in red and the protospacer adjacent motif (PAM) sequence in bold characters. Dashes and lower case letters indicate deleted and inserted bases, respectively (the number of inserted or deleted bases are described in the parentheses; out-of-frame and in-frame mutations are indicated using red and black colours, respectively). The number of occurrences is shown in parentheses; X1 and X2 indicates the number of each clone. Mutation frequencies were obtained by dividing the number of mutant clones by the number of total clones. Full size image When we tested this enrichment approach using BMP1 - and F13A1 -targeting RGENs, we observed mutation frequencies of 33 and 34%, respectively, after hygromycin selection, representing 12-fold and 5.6-fold enrichment of mutant cells (unselected cells displayed mutation frequencies of 2.8% and 6.1%, respectively) ( Fig. 7a,c ). This enrichment was corroborated by sequencing the genomic DNA around the target site, which revealed that the mutation frequency after transfection of plasmids encoding BMP1 and F13A1 -targeting RGENs was 6.7-fold (20%) and 7.3-fold (25%) higher, respectively, in the selected cells than in unselected cells ( Fig. 7b,d ). The mutation frequencies of cells transfected with only Cas9 and guide RNAs without the reporter plasmid, unselected cells at day 2 and unselected cells at day 4 after transfection were all comparable (in the PPP1R1B group, 6.6%, 6.4% and 6.6%, respectively; in the BMP1 group, 3.0%, 2.5% and 2.8%, respectively; in the F13A1 group, 6.9%, 5.8% and 6.1%, respectively), which are compatible with the observations using flow cytometric and magnetic reporters. Furthermore, hygromycin selection of HeLa cells revealed a 5.4-fold enrichment of cells containing RGEN-induced mutations ( Supplementary Fig. 8 ), indicating that the hygromycin system, like the flow cytometric and magnetic systems, is also applicable to other cell types. 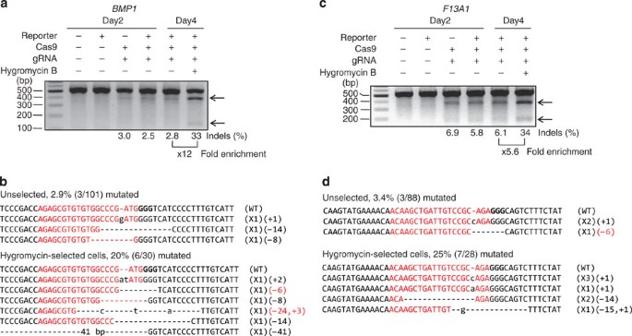Figure 7:Hygromycin selection-mediated enrichment ofBMP1- andF13A1-disrupted cells. HEK293T cells treated with hygromycin for 2 days starting 2 days after the cotransfection of the reporter plasmid, a plasmid encoding Cas9 and a plasmid encodingBMP1-(a,b) andF13A1-(c,d) targeting crRNA and tracrRNA. (a,c) The frequency of RGEN-induced mutations as determined by the T7E1 assay. Arrows indicate the expected positions of DNA bands cleaved by mismatch-sensitive T7E1. The numbers at the bottom of the gel indicate mutation percentages calculated by band intensities. (b,d) DNA sequences of the wild-type (WT) and mutant clones, with RGEN recognition sites shown in red and the protospacer adjacent motif (PAM) sequence in bold characters. Dashes and lower case letters indicate deleted and inserted bases, respectively (the number of inserted or deleted bases are described in the parentheses; out-of-frame and in-frame mutations are indicated using red and black colours, respectively). The number of occurrences is shown in parentheses; X1, X2 and X3 indicate the number of each clone. Mutation frequencies were obtained by dividing the number of mutant clones by the number of total clones. Figure 7: Hygromycin selection-mediated enrichment of BMP1 - and F13A1 -disrupted cells. HEK293T cells treated with hygromycin for 2 days starting 2 days after the cotransfection of the reporter plasmid, a plasmid encoding Cas9 and a plasmid encoding BMP1- ( a , b ) and F13A1- ( c , d ) targeting crRNA and tracrRNA. ( a , c ) The frequency of RGEN-induced mutations as determined by the T7E1 assay. Arrows indicate the expected positions of DNA bands cleaved by mismatch-sensitive T7E1. The numbers at the bottom of the gel indicate mutation percentages calculated by band intensities. ( b , d ) DNA sequences of the wild-type (WT) and mutant clones, with RGEN recognition sites shown in red and the protospacer adjacent motif (PAM) sequence in bold characters. Dashes and lower case letters indicate deleted and inserted bases, respectively (the number of inserted or deleted bases are described in the parentheses; out-of-frame and in-frame mutations are indicated using red and black colours, respectively). The number of occurrences is shown in parentheses; X1, X2 and X3 indicate the number of each clone. Mutation frequencies were obtained by dividing the number of mutant clones by the number of total clones. Full size image Comparison of reporters and enrichment methods In summary, the three different enrichment methods, each tested using three RGENs, enriched mutant cells from 3.7–11-fold (mean 7.7-fold, median 7.4-fold) ( Table 1 ). Interestingly, the fold enrichment tends to be high when RGEN activities are low ( Fig. 8a ), leading to comparable mutation frequencies that ranged from 20 to 33% (fold difference between the highest/lowest=1.7) after the selection; in comparison, the mutation frequencies before enrichment ranged from 2.8 to 7.1% (fold difference between the highest/lowest=2.6) ( Fig. 8b ). In our current experiments, the fold enrichments were similar among the three selection methods ( Fig. 8c ), which is also in line with previous studies using ZFNs and TALENs [27] . Thus, researchers can choose the reporter system that best fits their experimental conditions and research environment on the basis of previously described pros and cons of each reporter [27] . Table 1 Efficiencies of mutant cell enrichment using surrogate reporters. 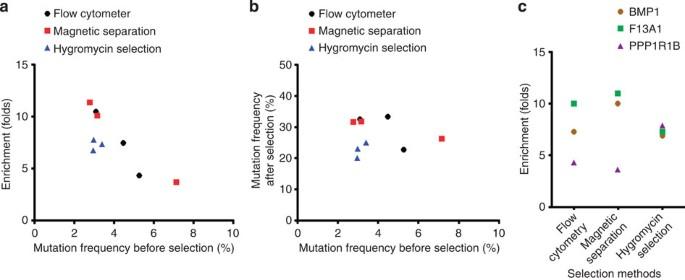Figure 8:Factors affecting fold enrichment. (a,b) The association of fold enrichment, mutation frequencies before selection and mutation frequencies after selection are shown. Mutation frequencies were calculated from sequencing results. Each dot represents an independent experiment. The selection methods used are symbolized with different coloured symbols. (c) The relationship between fold enrichment and selection method. Each dot represents an independent experiment. The targeted genes are symbolized using different coloured symbols. Full size table Figure 8: Factors affecting fold enrichment . ( a , b ) The association of fold enrichment, mutation frequencies before selection and mutation frequencies after selection are shown. Mutation frequencies were calculated from sequencing results. Each dot represents an independent experiment. The selection methods used are symbolized with different coloured symbols. ( c ) The relationship between fold enrichment and selection method. Each dot represents an independent experiment. The targeted genes are symbolized using different coloured symbols. Full size image Reporter cotransfection effects Our previous study using ZFNs showed that reporter-mediated selection results in the enrichment of highly transfected cells, which partially accounts for the enrichment of mutant cells [24] . To determine whether this phenomenon is true for RGENs, we sorted cells depending on RFP expression (an indicator of the level of transfection) and evaluated the mutation frequencies ( Supplementary Fig. 9 ). As expected, the T7E1 assay revealed that cells containing mutations were enriched in the following order: RFP bright (31% with mutations), RFP medium (24%) and RFP dim (9.2%), indicating that high levels of transfection can lead to high mutation frequencies. However, the degree of enrichment of gene-disrupted cells even in the RFP bright population was lower than that in the RFP + GFP + population (48%), suggesting that our reporter system is more useful for enrichment than simple sorting based on transfection efficiency alone, which is in line with our previous results using ZFNs [24] . We next determined whether the target sequence in the reporter plasmid competes with that in the genomic DNA, thereby attenuating the RGEN-induced editing of the genomic target sequence. We cotransfected various amounts of a reporter plasmid containing the target sequence together with a fixed amount of plasmid encoding an RGEN (targeting PPP1R1B ). To make the total amount of transfected DNA constant, we cotransfected compensating amounts of a reporter plasmid with a different target sequence (from the BMP1 gene in this case) from that of the RGEN. The T7E1 assay revealed that the efficiency of RGEN-induced gene disruption at the target sequence on the host chromosome was not changed by the transfection of a high amount of target sequence-bearing reporter plasmid ( Supplementary Fig. 10 ), suggesting that the presence of many copies of target sequence in the transfected reporter plasmid does not attenuate the creation of RGEN-induced gene mutations at the target sequence on the host chromosome. This conclusion is in line with our previous results showing that cotransfection of a target sequence-containing reporter plasmid does not affect the efficiency of ZFN- and TALEN-directed genome editing [24] , [27] . Out-of-frame mutation ratio and off-target effects We also determined the frequency of null (out-of-frame) versus in-frame mutations before and after enrichment. The frequency of out-of-frame mutations among total mutations ranged from 57 to 100% and was not changed significantly in nine independent enrichments ( Supplementary Table 1 ). The frequency of out-of-frame mutations that cause gene disruption among the total sequenced alleles ranged from 2.1–7.1% before enrichment and from 13–33% after enrichment, resulting in 2.6–11-fold enrichment of out-of-frame mutations, which is similar to enrichment folds of total mutations. Recently, it has been reported that RGENs can have off-target effects [29] , [30] , [31] , [32] , [33] , [34] , [35] . When we determined the mutation frequencies at the four to five top off-target sites of all three RGENs used in the study, we found that we did not detect off-target effects even after enrichment ( Supplementary Figs 11–13 ), raising the possibility that our enrichment process does not exacerbate off-target effects. Here we showed that cells containing RGEN-induced mutations can be enriched using flow cytometry, magnetic separation or hygromycin selection. Given that the fold enrichment tends to be higher when RGENs with low activity are used, our enrichment methods will be particularly useful when RGENs with high activity are not available; thus, these reporters complement RGENs so that RGENs coupled with reporters represent a reliable approach for making gene-disrupted cells. Partly because RGENs are easier and simpler to prepare in-house than ZFNs or TALENs, RGENs are expected to be used more widely as a genome-editing tool and to be preferred by beginners in genome editing. Such beginners would be more likely to design RGENs with low activity and/or to make mistakes in one or more genome-editing steps. Our reporters will be useful in this situation because they enable both monitoring of RGEN activity in live cells with fluorescent microscopy and the enrichment of genome-edited cells, a process that is more robust with low activity RGENs. Furthermore, in all three reporter systems, the enrichment process can also be monitored indirectly with fluorescent microscopy by evaluating the fraction of GFP + cells. We found that the addition of an episomal target sequence did not attenuate the RGEN-induced editing of the genomic target sequence. We tested a range of amounts of the reporter-incorporated episomal target sequence, up to ninefold higher than the ordinary amount of reporter (we could not evaluate the effect of adding even more reporters because the amount of DNA that can be transfected is limited). This lack of effect on RGEN activity suggests that the amount of guide RNA and Cas9 protein is sufficient to edit both the episomal and genomic target sequences within this tested range. This unaltered RGEN activity at the genomic target site is compatible with previous results [24] , [27] and is one of the practical advantages of our reporter system. RGENs are emerging as an approachable genome-editing tool. This is the first study showing that RGEN-induced mutations can be enriched using surrogate reporters. The three reporters resulted in comparable enrichment; researchers can choose a reporter system on the basis of their experimental conditions. We envision that these three types of reporters will facilitate the use of RGENs in a wide range of biomedical studies. Reporters Reporters were prepared as previously described [24] , [27] . Briefly, oligonucleotides including target sequences ( Supplementary Table 2 ) were synthesized (Bioneer, Daejon, South Korea) and annealed in vitro using a thermocycler (95 °C for 5 min and then ramped down to 25 °C at 5 °C per min). The annealed oligonucleotides were ligated into the reporter vectors digested with EcoR1 and BamH1. RGENs The Cas9-expressing p3s-Cas9HC plasmid has been previously described [4] and is available from Addgene (#43945). To construct the pRG2-CT plasmid, which expresses crRNA and tracrRNA under the control of the hU6 promoter, U6-crRNA and U6-tracrRNA cassettes were generated in the pLKO.1-puro plasmid and then sequentially subcloned into the minimal pUC18 backbone plasmid. The full sequence of this vector is described in Supplementary Fig. 14 and the vector map is shown in Supplementary Fig. 15 . Oligonucleotides containing each target sequences were synthesized (Macrogen, Seoul, South Korea) and annealed in vitro using a thermocycler. The pRG2-CT vector was digested with BsaI and ligated with annealed oligonucleotides. Oligonucleotide sequences are listed in Supplementary Table 3 . Cell culture Human embryonic kidney 293T (HEK293T) cells and HeLa cells (human cervical cancer cells) were purchased from American Type Culture Collection (Manassas, VA) and maintained in Dulbecco’s modified Eagle medium (DMEM; Invitrogen, Carlsbad, CA, USA) supplemented with 100 units ml −1 penicillin, 100 μg ml −1 streptomycin and 10% fetal bovine serum. Transfection Cells were transfected using lipofectamine 2000 (Invitrogen, Carlsbad, CA, USA) or polyethyleneimine (linear, MW~25,000; Polysciences, Warrington, PA, USA) at a weight ratio of 1:2:1 (plasmid encoding a Cas9: plasmid encoding crRNA and tracrRNA: reporter) unless specified otherwise. Flow cytometry Adherent cells were trypsinized and resuspended in 2% FBS in PBS. Single-cell suspensions were analysed and sorted using the FACSAria II cell sorter (BD Biosciences, San Jose, CA, USA). To collect cells that contain RGEN-induced mutations, cells with strong eGFP signals were sorted. Untransfected cells and cells transfected with reporters alone were used as controls. Magnetic separation Magnetic separations were performed as previously described [27] . Briefly, the transfected cells were cultured for 3 days and trypsinized. Cell suspensions were mixed with a magnetic bead-conjugated antibody against H-2K k (MACSelect K k microbeads; Miltenyi Biotech, Germany) at 80 μl antibody per 1 × 10 7 cells and incubated for 20 min at 4 °C. Labelled cells were separated using a column (MACS LS column; Miltenyi Biotech) according to the manufacturer’s instructions. Hygromycin selection Two days after transfection, hygromycin (Invitrogen, Carlsbad, CA, USA) was added to the culture media at a final concentration of 2 mg ml −1 for 2 days. T7E1 assay The T7E1 assay was performed as previously described [24] , [26] , [36] . Briefly, after the isolation of genomic DNA using the DNeasy Blood & Tissue Kit (Qiagen, Valencia, CA, USA) according to the manufacturer’s instructions, the region of DNA containing the nuclease target site was nested PCR-amplified using appropriate primers ( Supplementary Table 4 and 5 ). The amplicons were denatured by heating and annealed to form heteroduplex DNA, which was treated with 5 units of T7 endonuclease 1 (New England Biolabs) for 15–20 min at 37 °C and analysed using 2% agarose gel electrophoresis. Mutation frequencies were calculated as previously described based on the band intensities using Image J software and the following equation [37] : mutation frequency (%)=100 × (1−(1−fraction cleaved) 1/2 ), where the fraction cleaved is the total relative density of the cleavage bands divided by the sum of the relative density of the cleavage bands and uncut bands. Sequencing analysis Sequencing of the region including the target sequence was performed as previously described [24] , [27] . Briefly, PCR amplicons that included RGEN-target sites were cloned into the T-Blunt vector. Cloned plasmids were sequenced using the primers used for PCR amplification. How to cite this article: Ramakrishna, S. et al. Surrogate reporter-based enrichment of cells containing RNA-guided Cas9 nuclease-induced mutations. Nat. Commun. 5:3378 doi: 10.1038/ncomms4378 (2014).